Description and first application of a new technique to measure the gravitational mass of antihydrogen Physicists have long wondered whether the gravitational interactions between matter and antimatter might be different from those between matter and itself. Although there are many indirect indications that no such differences exist and that the weak equivalence principle holds, there have been no direct, free-fall style, experimental tests of gravity on antimatter. Here we describe a novel direct test methodology; we search for a propensity for antihydrogen atoms to fall downward when released from the ALPHA antihydrogen trap. In the absence of systematic errors, we can reject ratios of the gravitational to inertial mass of antihydrogen >75 at a statistical significance level of 5%; worst-case systematic errors increase the minimum rejection ratio to 110. A similar search places somewhat tighter bounds on a negative gravitational mass, that is, on antigravity. This methodology, coupled with ongoing experimental improvements, should allow us to bound the ratio within the more interesting near equivalence regime. There are many compelling experimental and theoretical arguments [1] , [2] , [3] , [4] , [5] , [6] , [7] , [8] , [9] , [10] that suggest that the gravitational mass of antimatter cannot differ from the gravitational or inertial mass of normal matter, that is, that the weak equivalence principle holds. For instance, one such argument comes from the absence of anomalies in Eötvös experiments conducted with differing atoms [4] ; the differing number of virtual particle–antiparticle pairs in such atoms might have caused gravitational anomalies to occur. However, all of these arguments are indirect and are not universally accepted [11] , [12] , [13] , [14] ; they rely on assumptions about the gravitational interactions of virtual antimatter, on postulates such as CPT invariance, or on other theoretical premises. Although these arguments may well be correct, in a world in which physicists have only recently discovered that we cannot account for most of the matter and energy in the universe, it would be presumptuous to categorically assert that the gravitational mass of antimatter necessarily equals its inertial mass. Moreover, the baryogenesis problem suggests that our understanding of antimatter is incomplete; gravitational asymmetries have been proposed as an explanation [7] , [15] , [16] . (Note that ref. 7 ultimately rejected gravity as a solution to the baryogenesis problem because of a thermodynamic proof of the weak equivalence principle. This proof was later challenged [10] .) There have not yet been any direct [14] , free-fall or gravitational balance, tests of the gravitational interactions of observable matter and antimatter. Direct gravitational experiments with non-neutral antimatter, for example, isolated positrons or antiprotons, are exceedingly difficult because the electrical forces overwhelm the gravitational forces [17] . Employing neutral antihydrogen [18] , [19] , [20] , [21] , [22] , [23] , [24] , [25] or positronium [26] eliminates this complication. The AEGIS project [27] at CERN was formed to conduct direct experimental tests of gravity on antihydrogen, and is now in its final construction phase. A second experiment, GBAR, has recently been approved at CERN [28] , and a third experiment was proposed at Fermilab [29] . This article describes a novel method that yields directly measured limits on the ratio of the gravitational to inertial mass of antimatter, accomplished essentially by searching for the free fall (or rise) of 434 ground-state antihydrogen atoms in the ALPHA [30] , [31] , [32] experiment at CERN. Our results set statistical bounds on the value of F ≡ M g / M , the ratio of the gravitational mass M g to the inertial mass M of antihydrogen. ( M is assumed numerically equal to the mass of hydrogen.) In the absence of systematic errors, we find that F must be <75 at a statistical significance level of 5%; worst-case systematic errors increase this limit to F <110. A similar search places somewhat tighter bounds on a negative F , that is, on antigravity. Refinements of our technique, coupled with larger numbers of cold-trapped anti-atoms, should allow us to bound F more tightly in future experiments and approach the | F |≈1 regime of widespread interest. Antihydrogen trapping ALPHA traps antihydrogen atoms by producing and capturing them in a minimum-B trap [33] . These traps confine those anti-atoms whose magnetic moment is aligned such that they are attracted to the minimum in the trap magnetic field B , and whose kinetic energy is below the trap well depth, . In ALPHA (see Fig. 1 ), this magnetic minimum is created by an octupole magnet that produces transverse fields of magnitude 1.54 T at the trap wall at R Wall =22.3 mm, and two mirror coils that produce axial fields of 1 T at their centres. The mirror coil centres are offset by ±138 mm from the trap centre. (The relative orientation of these coils and the trap boundaries are shown in Fig. 1 .) These fields are superimposed on a uniform axial field of 1 T produced by an external solenoid [34] , [35] . 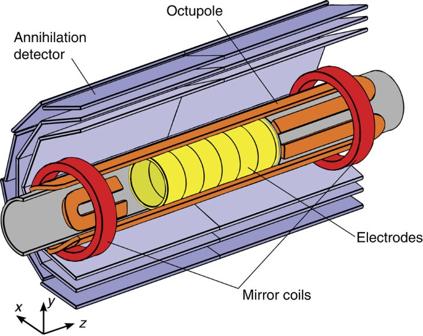Figure 1: Experimental schematic. A schematic, cut-away diagram of the antihydrogen production and trapping region of the ALPHA apparatus, showing the relative positions of the cryogenically cooled Penning-Malmberg trap electrodes, the minimum-B trap octupole and mirror magnet coils, and the annihilation detector. The trap wall is on the inner radius of the electrodes. Not shown is the solenoid, which makes a uniform field in. The components are not drawn to scale. Figure 1: Experimental schematic. A schematic, cut-away diagram of the antihydrogen production and trapping region of the ALPHA apparatus, showing the relative positions of the cryogenically cooled Penning-Malmberg trap electrodes, the minimum-B trap octupole and mirror magnet coils, and the annihilation detector. The trap wall is on the inner radius of the electrodes. Not shown is the solenoid, which makes a uniform field in . The components are not drawn to scale. Full size image The general methods by which anti-atoms are captured are described in refs 30 , 31 , 32 , 36 ; in this article we concentrate only on the last phase of the experiments, during which anti-atoms are released from the minimum-B trap by turning off the octupole and mirror fields. The escaping anti-atoms are then detected when they annihilate on the trap wall; a silicon-based annihilation vertex imaging detector [37] records the times (binned to 0.1 ms) and locations (azimuthal FWHM of 8 mm) of these annihilations. Annihilation time history on release The time history of the annihilations is critical to our analysis. This history is governed by the near-exponential decay of the octupole and mirror fields after the magnet turn-off is initiated. The fields decay with time constants of ∼ 9.5 ms ( [38] ). (Throughout this paper, times t are referenced to the initiation of the magnet shutdown.) At t =20 ms, for example, the maximum octupole field is ∼ 0.18 T and the mirror fields are ∼ 0.12 T. The trapping potential depth, which was originally ∼ 540 mK at t =0 ms, is reduced to ∼ 11 mK in the radial direction at t =20 ms. (Here we use kelvin as an energy unit.) Note that the 1 T solenoidal field, which is oriented parallel to the trap axis (the direction), is never varied. The well depth, which is proportional to the change in the magnitude of the total magnetic field as one progresses outwards from the trap centre, diminishes more slowly ( ∼ 80 mK at 20 ms) in the axial direction than in the radial direction. This is because the -directed mirror fields add linearly to the solenoidal field, while the - and -directed octupole fields add in quadrature to this field. Consequently, almost all of our trapped antihydrogen escapes radially [31] . Previous studies using the ALPHA apparatus have shown that the anti-atoms have a distribution in centre-of-mass energy ɛ that scales approximately like below the trapping threshold [31] , [38] . An anti-atom can escape the ever-shallower trap when its energy is greater than the trap depth. However, there is no one-to-one correspondence between the escape time of an anti-atom and its initial energy because it can take some time for an anti-atom to find the ‘hole’ in the trap potential. Computer simulations of this process, described in ref. 38 , show that anti-atoms of a given initial energy escape over a temporal range of at least 10 ms. The simulations discussed in ref. 38 did not include a gravitational force; to aid in our interpretation of the current experimental data, we extended these simulations to include gravity by the addition of a gravitational term to the equation of motion: where is the centre-of-mass position of the anti-atom, and g is the local gravitational acceleration. Previous measurements [39] on ALPHA established that the magnitude of the magnetic moment equals that of hydrogen to the accuracy required in this paper; its direction is assumed to adiabatically track the external magnetic field. Simulation studies To model the experiment, we simulated the effects of gravity on an ensemble of ground-state antihydrogen atoms randomly selected from the energy distribution described above. These anti-atoms are first propagated for 50 ms in the full-strength trap fields to effectively randomize their positions, and then propagated in the post-shutdown decaying fields until they annihilate on the trap wall. The results of a typical simulation are shown in Fig. 2 for F =100, which exaggerates the effects of gravity relative to the baseline of F =1 expected from the equivalence principle. As can be seen in Fig. 2 , there is a tendency for the anti-atoms to annihilate in the bottom half ( y <0) of the trap. This tendency is pronounced for anti-atoms annihilating at later times. This is because, as shown in Fig. 3 and in Table 1 , the confining potential well associated with the magnetic and gravitational forces in equation 1 is most skewed by gravitational effects late in time when the magnetic restoring force is relatively weak, and the remaining particles are those with the lowest energy. We note that while the number of late annihilating anti-atoms is dependent on the exact energy distribution used to initialize the simulations, the annihilation locations of these anti-atoms are not; for the purposes of this paper, the exact distribution is unimportant. 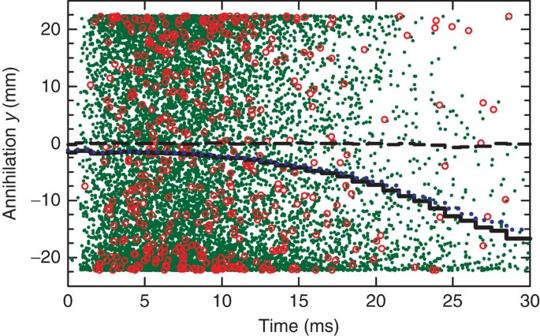Figure 2: Annihilation locations. The times and vertical (y) annihilation locations (green dots) of 10,000 simulated antihydrogen atoms in the decaying magnetic fields, as found by simulations of equation 1 withF=100. BecauseF=100 in this simulation, there is a tendency for the anti-atoms to annihilate in the bottom half (y<0) of the trap, as shown by the black solid line, which plots the average annihilation locations binned in 1 ms intervals. The average was taken by simulating approximately 900,000 anti-atoms; the green points are the annihilation locations of a sub-sample of these simulated anti-atoms. The blue dotted line includes the effects of detector azimuthal smearing on the average; the smearing reduces the effect of gravity observed in the data. The red circles are the annihilation times and locations for 434 real anti-atoms, as measured by our particle detector. Also shown (black dashed line) is the average annihilation location for∼840,000 simulated anti-atoms forF=1. Figure 2: Annihilation locations. The times and vertical ( y ) annihilation locations (green dots) of 10,000 simulated antihydrogen atoms in the decaying magnetic fields, as found by simulations of equation 1 with F =100. Because F =100 in this simulation, there is a tendency for the anti-atoms to annihilate in the bottom half ( y <0) of the trap, as shown by the black solid line, which plots the average annihilation locations binned in 1 ms intervals. The average was taken by simulating approximately 900,000 anti-atoms; the green points are the annihilation locations of a sub-sample of these simulated anti-atoms. The blue dotted line includes the effects of detector azimuthal smearing on the average; the smearing reduces the effect of gravity observed in the data. The red circles are the annihilation times and locations for 434 real anti-atoms, as measured by our particle detector. Also shown (black dashed line) is the average annihilation location for ∼ 840,000 simulated anti-atoms for F =1. 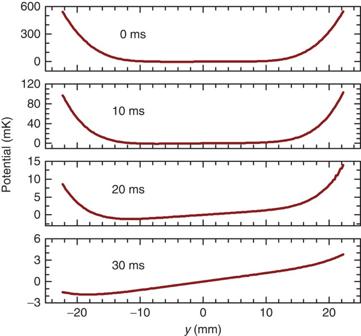Figure 3: Potential well. The potential well, forF=100, at the indicated times and atz=0. The flat-bottomed appearance of the well at early times results from the quadratic addition of the solenoidal field to ther3dependent octupole field. (Here,ris the transverse radius.) Full size image Figure 3: Potential well. The potential well, for F =100, at the indicated times and at z =0. The flat-bottomed appearance of the well at early times results from the quadratic addition of the solenoidal field to the r 3 dependent octupole field. (Here, r is the transverse radius .) Full size image Table 1 Trap depths. Full size table Reverse cumulative average analysis To determine an experimental limit on F , we compare our data set of 434 observed antihydrogen annihilation events to computer simulations at various F ’s. Our statistics suffer from the fact that escaping anti-atoms are most sensitive to gravitational forces at late times, but relatively few of the events occur at late times. For example, even with the cooling due to the adiabatic expansion that occurs as the trap depth is lowered, only 23 anti-atoms out of the 434 annihilate after 20 ms. Moreover, inspection of the simulation data in Fig. 2 shows that even when there is a pronounced tendency for the anti-atoms to fall down, some still annihilate near the top of the trap. To obtain a qualitative understanding of the data, we use the reverse cumulative average 〈 y | t 〉: the average of the y positions of all the annihilations that occur at time t or later (see Methods). This reverse cumulative average highlights the more informative late-time events while still including as many events as possible into the average. 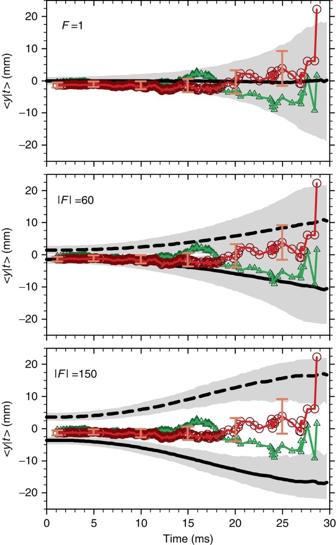Figure 4: Reverse cumulative average analysis. Comparison of the reverse cumulative average 〈y|t〉 of the event data to the reverse cumulative average of the simulation data. Each plot is identified by the value ofFused in the simulations. In all graphs, the red-circle line is the 〈y|t〉 of theyannihilation positions of the event data. The green-triangle line is the reverse cumulative average of thexannihilation positions of the event data, and is included as a comparison. The black solid line is the 〈y|t〉 of approximately 900,000 simulated antihydrogen atoms. The black dashed line mirrors the black-solid line around 〈y|t〉=0, and is equivalent to a simulation study of antigravity, i.e., negativeF. The grey bands demark the 90% confidence region (95% when interpreted as a one-sided confidence test) for 434 annihilations around the gravity and antigravity 〈y|t〉. The procedures for computing the 〈y|t〉 and the error bands are described in the Methods. The error bars on the event data give the standard error of the mean for 〈y|t〉. The calculated lines do not include the effects of systematic errors. Figure 4 plots 〈 y | t 〉 for the events and the simulations at several values of F . These plots suggest that an upper bound on F can be established from the data, at a value somewhere between F =60 and 150. Figure 4: Reverse cumulative average analysis. Comparison of the reverse cumulative average 〈 y | t 〉 of the event data to the reverse cumulative average of the simulation data. Each plot is identified by the value of F used in the simulations. In all graphs, the red-circle line is the 〈 y | t 〉 of the y annihilation positions of the event data. The green-triangle line is the reverse cumulative average of the x annihilation positions of the event data, and is included as a comparison. The black solid line is the 〈 y | t 〉 of approximately 900,000 simulated antihydrogen atoms. The black dashed line mirrors the black-solid line around 〈 y | t 〉=0, and is equivalent to a simulation study of antigravity, i.e., negative F . The grey bands demark the 90% confidence region (95% when interpreted as a one-sided confidence test) for 434 annihilations around the gravity and antigravity 〈 y | t 〉. The procedures for computing the 〈 y | t 〉 and the error bands are described in the Methods. The error bars on the event data give the standard error of the mean for 〈 y | t 〉. The calculated lines do not include the effects of systematic errors. Full size image Monte Carlo analysis Although the visual approach taken in Fig. 4 is striking, a more sophisticated analysis is necessary for a quantitative assessment of F . Specifically, our problem is this: given our event set of experimental annihilations {( y , t )} Ev , where y is the observed position of a given annihilation and t is the time of this annihilation, and given a family of similar sets of simulated pseudo-annihilations {( y , t )} F at various F , how can we determine which values of F can be excluded with reasonable confidence? In other words, which sets {( y , t )} F are unlikely to be compatible with {( y , t )} Ev ? (In this paper, the phrase ‘pseudo-annihilations’ or ‘pseudo-events’ always refers to simulation results. The unqualified word ‘events’ always refers to experimental results.) We make this determination with a Monte Carlo analysis based on an overall test statistic, that is, a figure-of-merit, Φ, which is sensitive to discrepancies between the real and simulated data. Our choice of Φ is closely related to a Fisher’s combined test [40] based on Kolmogorov-Smirnov (K-S) [41] statistics. The exact definition of Φ is described in the Methods section. In brief, for every F , we calculate the test statistic Φ Ev for the experimental events. This Φ Ev compares {( y , t )} Ev to a reference distribution compiled from a third ( ∼ 300,000 simulated annihilations) of the simulation data set {( y , t )} F . The test statistic Φ is small when it is likely that the 434 events could have been drawn from the reference distribution, and large when it is unlikely that the events could have been so drawn, that is, when there is a significant disparity between the distribution of the actual events and the reference distribution of the simulated annihilations at the hypothesized F . Next, to approximate the sampling distribution for Φ, we distribute the remaining pseudo-annihilations in {( y , t )} F into N pseudo-event subsets of 434 points. In total there are about 900,000 pseudo-events in {( y , t )} F , so N is about 1,400. Each of these pseudo-event sets is representative of what we would have observed if the ratio of the inertial to the gravitational mass really was F . Then, we calculate the set of test statistics {Φ i ; F } for each of these pseudo-event sets, and count the number N > for which Φ i ; F ≥Φ Ev , that is, the number of pseudo-event sets that are less compatible with the reference distribution than the actual events. From N > , we obtain a Monte Carlo estimate of the overall P -value, P = N > / N , for the goodness-of-fit test on the actual data set compared with the simulations. The results of this analysis are shown in Fig. 5 , from which we conclude that F >75 is excluded at a significance level of 5%. 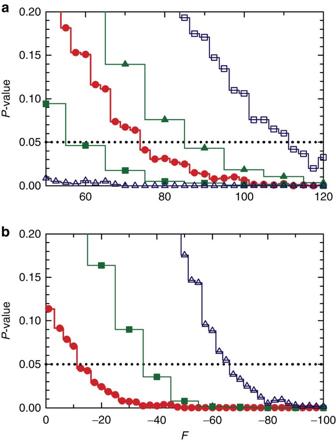Figure 5: Monte Carlo analysis. EstimatedP-values for the combined test statistic Φ as a function ofFfor (a) gravitational interactions (F>0), and (b) anti-gravitational interactions (F<0). The probabilities are computed using a Monte Carlo study of the Fisher combined statistic, as discussed in the Methods. The red solid circle lines assume no systematic errors; the blue hollow square line assumes a detector displacement of −5 mm; the green solid triangle line assumes an octupole axis displacement of +0.05 mm; the green solid square lines assume an octupole axis displacement of −0.05 mm; the blue hollow triangle lines assume a detector displacement of +5 mm. (For (b), theP-values for a detector displacement of −5 mm or for an octupole axis displacement of +0.05 mm are essentially zero.) These four systematic errors encompass the range allowed by mechanical constraints. Figure 5: Monte Carlo analysis. Estimated P -values for the combined test statistic Φ as a function of F for ( a ) gravitational interactions ( F >0), and ( b ) anti-gravitational interactions ( F <0). The probabilities are computed using a Monte Carlo study of the Fisher combined statistic, as discussed in the Methods. The red solid circle lines assume no systematic errors; the blue hollow square line assumes a detector displacement of −5 mm; the green solid triangle line assumes an octupole axis displacement of +0.05 mm; the green solid square lines assume an octupole axis displacement of −0.05 mm; the blue hollow triangle lines assume a detector displacement of +5 mm. (For ( b ), the P -values for a detector displacement of −5 mm or for an octupole axis displacement of +0.05 mm are essentially zero.) These four systematic errors encompass the range allowed by mechanical constraints. Full size image A similar Monte Carlo analysis comparing the actual event data to F =1 simulations gives an unsurprising overall P -value of 0.3. Thus, the event data are not incompatible with F =1, but we cannot conclude that F ≈1. Systematic error analysis In the ∼ 800 trapping trials used to obtain our 434 point event set, we would expect approximately one cosmic ray to be misclassified as an antihydrogen atom [30] , [32] . Thus, cosmic rays are an insignificant source of error in this analysis. The cosmic ray background does, however, preclude our using annihilation data from times later than 30 ms, as the current data rate would not be comfortably above the cosmic rate at such late times. Previously, we calculated [31] that more than 99.5% of antihydrogen atoms held longer than 400 ms will have decayed to the ground state. The 434 trapped anti-atoms employed in the analysis were all held for times longer than this. Thus, we expect that virtually all of our anti-atoms are in the ground state, and are largely immune to Stark effect/polarization forces that might have otherwise overwhelmed the gravitational forces. The largest electric fields in our trap during the magnet shutdown phase come from the ‘bias’ potential that we use to discriminate between antihydrogen atoms and antiprotons [30] , [31] , [38] and exist in the 0.75-mm gap between the electrodes. These fields are on the order of 10 V mm −1 . The energy that a ground-state antihydrogen atom would acquire approaching this gap is about five orders of magnitude less than the F =1 gravitational potential drop across the trap diameter. Furthermore, such a high field exists only in a very small volume of the trap. The ‘patch’ fields [17] that plague charged particle gravity tests perturb the anti-atom energy by about two orders of magnitude less than the bias electric fields. The annihilation detection algorithm determines the locations of the anti-atom annihilations from the tracks of the pions that result from each annihilation. The smearing that results from the limited spatial resolution of the detector is well characterized [37] and is incorporated into our analysis (see Methods). The largest uncertainty in limiting F comes from our neglect, up to this point, of systematic effects from mechanical misalignments and from magnetic field errors. For example, the detector might not be perfectly centred on the trap axis. This misalignment is limited by mechanical constraints to be no more than ±5 mm. Such a misalignment would cause an apparent shift in the annihilation locations at early times as well as late, resulting in a bias in the average of the entire event set, 〈 y | t =0〉, of ±2.5 mm if at the constraint limit. (These errors differ from the detector smearing errors, which were calculated assuming that the detector was perfectly centred.) A somewhat smaller error would result from the octupole axis being displaced from the trap axis, which would cause a shift in the real annihilation locations. Like the detector displacement error, this displacement would cause a bias in overall average 〈 y | t =0〉. A bias of unknown origin is indeed visible in the event data: 〈 y | t =0〉=−1.3±0.8 mm. Simulations incorporating an octupole axis displacement show that this overall bias would correspond to a axis displacement of only −0.06 mm. Perhaps coincidentally, this is nearly identical to the maximum displacement allowed by mechanical constraints. We have performed a broad survey (see Supplementary Note 1 ) of other magnetic field errors consistent with the mechanical tolerances of our device. This survey shows that the largest biases that could result from magnetic errors are usually smaller than, and at worst comparable to, the largest bias possible from an octupole axis displacement. Thus, in the absence of fortuitous cancelations, the relatively small measured bias in 〈 y | t =0〉 limits the size of the effects of these errors at the late times when the experiment is most sensitive to gravity. Taking the maximally allowed detector and octupole displacement errors as representative of the worst-case systematic errors, we have modelled their effects in the statistical calculations and, as shown in Fig. 5 , determined that the worst-case exclusion region is F >110, still at a significance level of 5%. Similarly, analysis of favourable systematic errors, say because of a fortuitous octupole axis displacement of −0.05 mm that would eliminate the 〈 y | t =0〉 bias, yields a best case exclusion of F >65 based on statistics alone. Some perspective on the size of the systematic errors can be found by calculating 〈 y | t =0〉 for the untrapped antihydrogen atoms and antiprotons that annihilate on the wall during the antihydrogen synthesis process. In an observed sample of over 270,000 of such anti-atoms, the y mean was +0.86±0.03 mm. However, the orbital dynamics of untrapped antihydrogen and antiprotons are quite different from the dynamics of trapped antihydrogen, and there are effects that can lead to average vertical displacements of the opposite sign. A Monte Carlo simulation of our detector, which includes the effects of dead regions, gives a mean value for y of +0.01±0.06 mm. A hitherto unutilized experimental sample of 120 trapped antihydrogen atoms had a y mean of +2.2±1.4 mm. (This sample was not otherwise utilized because the atoms in this sample could not be guaranteed to have been trapped for more than 400 ms. Hence, these atoms were not necessarily in the ground state [31] .) These means do not entirely reconcile with each other or with the y mean of the standard sample of trapped atoms (−1.3±0.8 mm), and we have no certain explanation of their differences. However, the range of means predicted by our analysis of the detector axis displacements encompasses all these values; thus, we allow for larger errors in our worst-case analysis. We set a limit on antigravity by inverting the sign of g in equation 1, or, equivalently, by making F negative. We find that F <−12 is excluded by statistics alone, with a worst-case limit from systematic errors of F <−65. However, because the systematic effects are not very well characterized for such small | F |, it is more conservative to only exclude F <−65. Importance of detailed studies of the orbital dynamics We stress that our determination of F relies on detailed simulations of anti-atom trajectories in the time-dependent trap magnetic fields; other gravitational measurements using trapped antihydrogen would likely require a similar analysis. A recent publication, ref. 42 , briefly mentions an experimental bound on F of 200. So far as we can discern from the one-paragraph description of the experiment, the measurement implicitly assumes thorough dynamical mixing between the transverse and axial directions. Previous antihydrogen simulations [31] , [38] show that these two directions are poorly coupled. This is because the trapping potential is nearly separable, and approximate independent constants of the motion exist for the transverse and axial degrees-of-freedom. Mixing only occurs due to end effects from the finite axial length of the magnetic system or from large size, small-spatial-scale magnetic errors unlikely to be present. Indeed, analytic calculations show that these constants of motion are adiabatically conserved for a broad range of parameters [43] . Furthermore, experiments [44] on the evaporative cooling of hydrogen atoms—a procedure closely analogous to the procedure outlined in ref. 42 —show that the evaporation is essentially one dimensional, not three; that is, the transverse and axial directions do not couple. Thus, it is not surprising that simulations based on the best model we can construct from the limited information available in ref. 42 show that no effects of gravity could be observed using the techniques described in ref. 42 for | F |≤200, or indeed, for | F |’s significantly greater than 200 (ref. 45 ). We report directly measured limits on the ratio of the gravitational mass to the inertial mass of antimatter. On the basis of goodness-of-fit tests comparing the positions of actual and simulated annihilation events, we can rule out ratios above F =75 (statistics alone) and F =110 (including worst-case systematic effects) for gravity, and below F =−65 (combined systematic and statistical effects) for antigravity, at the 5% significance level. Obviously, our limits are far from the F =1 regime where one could test for small deviations from the weak equivalence principle, but the methodology described here, coupled with planned and ongoing improvements to the ALPHA apparatus, should allow us to improve the measurement substantially. Simulations show that by cooling the anti-atoms, perhaps with lasers, to 30 mK or lower, and by lengthening the magnetic shutdown time constant to 300 ms, we would have the statistical power to measure gravity to the F =±1 level (see Fig. 6 ). Cooling obviously increases the relative influence of gravity on the anti-atom trajectories. The longer shutdown times are necessary to take full advantage of adiabatic expansion cooling of these slower anti-atoms. They also allow the anti-atoms to find and annihilate on the portions of the trap wall where the trapping well depth is lowest. Systematic errors pose a significant challenge for low F measurements, however, and will need to be addressed. In summary, our experiments are an important first step towards a precise gravitational measurement with trapped, neutral antimatter. The current work clearly demonstrates the potential for using a carefully prepared, well-characterized sample of trapped antihydrogen atoms as a source for direct, ballistic studies of the gravitational behaviour of antimatter. The use of untrapped neutral antimatter for gravitational measurements, as pursued by other groups [27] , [28] , is, as yet, unproven. 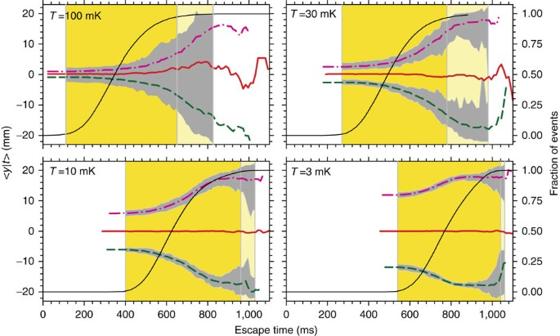Figure 6: Cooled antihydrogen analysis. The reverse cumulative averages 〈y|t〉 for antihydrogen atoms cooled to the temperaturesTlisted in each graph. The magnet shutdown has been slowed by a factor of ten. The magenta dash-dot line is forF=−1, the red solid line is forF=0, and the green dashed line is forF=+1. The dark yellow vertical band indicates the region in which the signal-to-cosmic-noise ratio (S/N) exceeds 5 for the current trapping rate31, and the light yellow vertical band indicates this same region (S/N>5) for an antihydrogen trapping rate ten times greater. The grey bands demark the 90% confidence region (95% when interpreted as a one-sided confidence test) for 500 annihilations around the gravity and antigravity 〈y|t〉; for simplicity, these bands are not plotted forF=0, and are only plotted within the regions of the high S/N bands. The thin black solid line shows the fraction of anti-atoms that have escaped as a function of time. Only counting statistics and signal-to-cosmic-noise effects are included in this graph; systematic effects at lowFneed to be further investigated. Figure 6: Cooled antihydrogen analysis. The reverse cumulative averages 〈 y | t 〉 for antihydrogen atoms cooled to the temperatures T listed in each graph. The magnet shutdown has been slowed by a factor of ten. The magenta dash-dot line is for F =−1, the red solid line is for F =0, and the green dashed line is for F =+1. The dark yellow vertical band indicates the region in which the signal-to-cosmic-noise ratio (S/N) exceeds 5 for the current trapping rate 31 , and the light yellow vertical band indicates this same region (S/N>5) for an antihydrogen trapping rate ten times greater. The grey bands demark the 90% confidence region (95% when interpreted as a one-sided confidence test) for 500 annihilations around the gravity and antigravity 〈 y | t 〉; for simplicity, these bands are not plotted for F =0, and are only plotted within the regions of the high S/N bands. The thin black solid line shows the fraction of anti-atoms that have escaped as a function of time. Only counting statistics and signal-to-cosmic-noise effects are included in this graph; systematic effects at low F need to be further investigated. Full size image Simulations Antihydrogen trajectories were simulated using codes developed to establish that ALPHA trapped antihydrogen [38] . The codes use an adaptive Runge-Kutta stepper to propagate antihydrogen atoms in the magnetic and gravitational fields of the trap. The model for the spatial structure and temporal behaviour of the magnetic field was experimentally verified by studying the trajectories of antiprotons [38] . (Also see Supplementary Note 2 .) The numeric value of the antihydrogen magnetic moment used in the simulations was set equal to that of the positron alone; the small deviations to the antihydrogen magnetic moment from the antiproton are not significant for the experiments reported here. As described previously, the simulations are initiated with anti-atoms with a random energy consistent with a distribution. Anti-atoms with energies up to 650 mK, well above the nominal trapping depth of ∼ 540 mK, are included. Most of the anti-atoms with energy above 540 mK are lost during the 50 ms randomization period before the magnet shutdown is initiated, but some, those on quasitrapped orbits [31] , [38] , [46] , are retained. The gravity analysis is almost independent of the exact distribution of these quasitrapped anti-atoms, however, because they are lost at very early t . Spatially, the simulations were initiated with anti-atoms that originate in a region mimicking the dimensions of the experimental positron plasma. The 50 ms randomization period is sufficient to distribute these anti-atoms within the trap [38] , but may not entirely randomize them. To look for effects of insufficient randomization, simulations were also run with randomization times of 1 and 10 s. Some differences were observed, but these differences were significantly smaller than the differences caused by the detector displacement errors discussed above. We note that almost 75% of the anti-atoms used in this analysis were held for times between 0.4 and 1.4 s, so the 1-s simulations model the approximate entire lifetime of the majority of the anti-atoms. Antihydrogen energy distribution To model the behaviour of anti-atoms during the magnet shutdown, we need to know the initial antihydrogen velocity distribution. ALPHA synthesizes antihydrogen atoms by injecting antiprotons into a positron plasma. The positron plasma is typically at a temperature of ∼ 40 K ( [30] ); before antihydrogen forms, the antiprotons thermalize on the positrons, giving them a temperature that approaches 40 K 47 . The resultant antihydrogen inherits the centre-of-mass kinetic energy of the antiprotons from which they are formed, so it too has an initial temperature of about 40 K. Most of these antihydrogen atoms are far too energetic to be trapped; only those with an energy near or below the trapping depth of 540 mK are sufficiently cold to be trapped. These trapped anti-atoms are deep within the Maxwellian distribution, where the energy distribution scales like . Strong evidence that the true energy distribution is close to this comes from comparing the annihilation times of the actual anti-atoms with the annihilation times of simulated anti-atoms for several different distributions (see Fig. 7a ). This comparison is shown in Fig. 7b , where it is clear that the Maxwellian distribution best fits the experimental events. However, there are some differences between the two; for example, the simulations slightly underpredict the number of late annihilating anti-atoms. Fortunately, the analysis is not very sensitive to the details of the distribution, so the small deviations from Maxwellian visible in Fig. 7b are unimportant. For instance, Fig. 7c shows the annihilation locations for anti-atoms that annihilate between 20 and 22 ms, and the differences between the three distributions plotted are barely discernible. 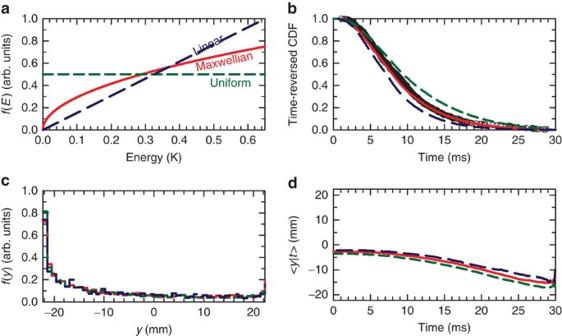Figure 7: Energy distribution analysis. The effect on the annihilation location for (a) three postulated initial energy distributions. As the trap depth is about 540 mK, most, but not all, of the anti-atoms beyond 540 mK will be untrapped31,38. (b) TheF=1 time-reversed CDF of the simulated annihilations during the magnet shutdown for the three distributions, following the labelling in (a). The black points plot the time-reversed CDF of the experimental events (which mainly appear as a band behind the red Maxwellian line.) The event data agrees well with the Maxwellian distribution. (c) A typical distribution inyof late annihilations (those occurring between 20 and 22 ms). (d) The reverse cumulative average, 〈y|t〉, for the three distributions, as defined in the text. For (c) and (d),F=80; as expected, the plotted lines in these last two graphs show little dependence on the postulated energy distribution. Figure 7d shows the influence of the choice of distribution on the reverse cumulative average 〈 y | t 〉, and the differences are also small. Figure 7: Energy distribution analysis. The effect on the annihilation location for ( a ) three postulated initial energy distributions. As the trap depth is about 540 mK, most, but not all, of the anti-atoms beyond 540 mK will be untrapped [31] , [38] . ( b ) The F =1 time-reversed CDF of the simulated annihilations during the magnet shutdown for the three distributions, following the labelling in ( a ). The black points plot the time-reversed CDF of the experimental events (which mainly appear as a band behind the red Maxwellian line.) The event data agrees well with the Maxwellian distribution. ( c ) A typical distribution in y of late annihilations (those occurring between 20 and 22 ms). ( d ) The reverse cumulative average, 〈 y | t 〉, for the three distributions, as defined in the text. For ( c ) and ( d ), F =80; as expected, the plotted lines in these last two graphs show little dependence on the postulated energy distribution. Full size image Reverse cumulative average The reverse cumulative average is formally defined to be 〈 y | t 〉=(1/ N t )Σ n y n , where { y n } is the set of annihilation locations, and the sum is over all of the N t elements of { y n } that occur after time t and before the late cutoff at 30 ms used to exclude the cosmic ray background. In Fig. 4 , 〈 y | t 〉 is shown for both the event data and the simulation data at the given F ’s. The Monte Carlo error bands in Fig. 4 are calculated by dividing the ∼ 900,000 point simulation set at given F into about 2,100 subsets of length 434—the size of the actual event sample. Then, at every t , 〈 y | t 〉 is calculated for each subset and the results ordered. The error band at every t is then defined by the 5 and 95% quantiles of the ordered 〈 y | t 〉. Detector resolution The detector determines the locations of the anti-atom annihilations by triangulation of the pion tracks produced by each annihilation. This process was extensively studied using the GEANT3 code [48] , and a probability density function for the azimuthal resolution error was determined [37] . This error was incorporated into the simulation results by adding random angular offsets consistent with this probability density function to each of the simulated annihilation angular locations. Statistical analysis To find the probability that the events are compatible with the simulations at a given F , we employ a test statistic akin to Fisher’s combined statistic [40] aggregating K-S tests in different (overlapping) time windows: where P KS ( t ; F ) is the approximate P -value for a one-sided, two-sample K-S test [41] , [49] for a given F . The K-S test, described in the next paragraph, indicates how compatible the y annihilation distribution of a specific trial data set, windowed between t and 30 ms, is with the y annihilation distribution of a similarly windowed reference data set. Specifically, at every F we extract a ∼ 300,000 point subset from the simulation data to serve as a reference data set. Then we compute P KS ( t ; F ) at every start time t and integrate using a numerical quadrature rule with a fixed time increment of 0.3 ms. Carrying out this procedure using the event data set for the trial distribution, we get the Φ Ev defined earlier. Carrying out this identical procedure using the remaining N ≈1,400 pseudo-event sets as the trial distributions, we get the set {Φ i ; F }. Under the null hypothesis, namely, that there is no difference between the distributions for a given F , the P KS ( t ; F ) themselves should be uniformly distributed. As originally introduced, Fisher’s combined test statistic was intended for independent tests, for which the overall P -value is χ 2 distributed. In our case, the K-S P -values are correlated in t because the t windows overlap, so the P -value of the combined test statistic is estimated by Monte Carlo sampling. Thus, P = N > / N , where the integer N > counts the number of Φ i , F for which Φ i , F >Φ Ev . For each time window and F , the K-S test computes a ‘distance’ between the cumulative distribution function (CDF) for y for a trial event or pseudo-event set, and a reference distribution CDF. A greater distance reflects a lower probability that samples drawn from the reference set could deviate from the ‘average’ of that set by more than the trial set. These distances translate to approximate K-S P -values, P KS ( t ; F ), through a well-studied universal function [49] , [50] . As our reference CDFs are rigorously stochastically ordered, yielding strictly declining P KS ( t ; F ) for increasing F ( t held fixed) once P is small, we can employ a one-sided K-S test rather than the more typical two-sided test. When the number of samples between t and 30 ms in the trial set, k is greater than 4, we use the standard asymptotic expansion [49] for the distance to P KS function; for smaller k we use the direct small-sample formulae. The P KS for small k are generally close to unity, and contribute little to Φ. The estimated P KS include ‘two-sample’ corrections to account for the sampling error in the reference CDFs; however, these corrections are very small because the simulation sample sizes are large. Any approximations involved in calculating the P KS do not greatly affect the overall P -value, as the former are not interpreted directly in terms of Type I (false positive) errors, but are only used to compute the combined test statistic Φ whose P -value is determined by Monte Carlo methods. Note that for the analysis of the compatibility of the events with F =1, which yielded an overall P -value of 0.3, the K-S P -values are not small and the use of the one-sided K-S test is not justified. Hence, in this case only, we used the two-sided K-S test. We have approached the statistical analysis from the perspective of significance testing, that is, by seeking to reject hypotheses corresponding to sufficiently large values of | F | for which the data appear incompatible. If desired, however, the unrejected interval, −65< F <110, which includes systematic errors, could also be interpreted as a confidence region for F (with a coverage probability of 95% corresponding to our 5% significance level). Event data set The event data set analysed here includes all those antihydrogen atoms trapped in the ALPHA apparatus in 2010 and 2011 that were held for more than 400 ms, escaped the trap within 30 ms of the magnet shutdown initiation, and whose annihilation locations reconstructed to be within z =±138 mm of the trap centre. Regions beyond z =±138 mm were excluded because the trap wall has a significant inward step at these z locations. How to cite this article: The ALPHA Collaboration and Charman, A.E. Description and first application of a new technique to measure the gravitational mass of antihydrogen. Nat. Commun . 4:1785 doi: 10.1038/ncomms2787 (2013).